Solar-induced direct biomass-to-electricity hybrid fuel cell using polyoxometalates as photocatalyst and charge carrier The current polymer-exchange membrane fuel cell technology cannot directly use biomass as fuel. Here we present a solar-induced hybrid fuel cell that is directly powered with natural polymeric biomasses, such as starch, cellulose, lignin, and even switchgrass and wood powders. The fuel cell uses polyoxometalates as the photocatalyst and charge carrier to generate electricity at low temperature. This solar-induced hybrid fuel cell combines some features of solar cells, fuel cells and redox flow batteries. The power density of the solar-induced hybrid fuel cell powered by cellulose reaches 0.72 mW cm −2 , which is almost 100 times higher than cellulose-based microbial fuel cells and is close to that of the best microbial fuel cells reported in literature. Unlike most cell technologies that are sensitive to impurities, the cell reported in this study is inert to most organic and inorganic contaminants present in the fuels. With the depletion of fossil energy and growing environmental concerns, developing renewable energy sources becomes more and more important [1] . Today, fossil fuels still dominate the energy market, accounting for 87% of global energy consumption [2] . Solar energy and biomass energy are two important sustainable energy sources [3] . Therefore, production of electricity to power our world from solar energy and biomass can reduce the dependence on fossil fuels. Biomass-to-electricity conversion using natural biomass resources can be realized by two common technologies: solid oxide fuel cells [4] , [5] , [6] and microbial fuel cells [7] , [8] . However, several critical issues exist with the current technologies. Solid oxide fuel cells require very high working temperatures (500~1,000 °C) for gasification of biomass [9] , [10] . Although microbial fuel cells can work at low temperature, very low electric power output, rigorous reaction conditions and limited lifetime seriously hinder their applications [11] , [12] . The polymer-exchange membrane fuel cell (PEMFC) is another most promising fuel cell technology. Although highly effective PEMFCs powered by hydrogen or low molecular weight alcohols have been successfully commercialized, polymeric biomass such as starch, lignin and cellulose have not been directly used in PEMFC because the C–C bonds cannot be completely electro-oxidized to CO 2 at low temperatures with a noble metal catalyst [13] , [14] . Even for the simplest C–C molecules such as ethanol, it was reported that the fuel could only be converted to acetaldehyde (−2e − ) or acetic acid (−4e − ) with a noble metal anode, suggesting that only 16.7 and 33.3% of the total 12 electrons can be actually converted to electric power [15] , [16] . Therefore, cleavage of C–C bonds in biomass fuels is a major challenge in developing high-efficiency PEMFCs. Furthermore, it is well known that noble metals such as Pt, Au, Ru and so on are easily poisoned by impurities in the biomass. For these reasons, a low-temperature PEMFC that directly uses natural polymeric biomasses has not been reported. Here we present a solar-induced hybrid fuel cell that directly consumes natural polymeric biomass, such as starch, lignin, cellulose, and even switchgrass or wood powders. With this hybrid fuel cell technology, the biomass is oxidized by polyoxometalates (POMs) in the solution under solar irradiation and the reduced POM is oxidized by oxygen through an external circuit, producing electricity. The designed solar-induced biomass hybrid fuel cell has many advantages. First, the cell combines photochemical and solar–thermal biomass degradation in a single chemical process, leading to high solar conversion and effective biomass degradation. Second, it does not use expensive noble metals as anode catalysts because the fuel oxidation reactions are catalysed by POMs in the solution rather than by noble metals on the anode electrode. Finally, the solar-induced hybrid fuel cell is directly powered by unpurified polymeric biomasses that could significantly reduce the fuel cell cost. Electron and proton transfer under photo-irradiation The structure of the solar-induced hybrid fuel cell is shown in Fig. 1 . It includes a common fuel cell equipped with a membrane electrode assembly (MEA) and a transparent glass fuel storage vessel that can be pre-irradiated with light. It should be noted that the cathode electrode included Pt (60%)/C catalyst (5 mg cm −2 ), but the anode electrode was made of simple carbon cloth without Pt. Experimentally, the biomass–POM electrolyte solution was either pre-irradiated before circulation in the anode cell or irradiated in situ to generate electricity. 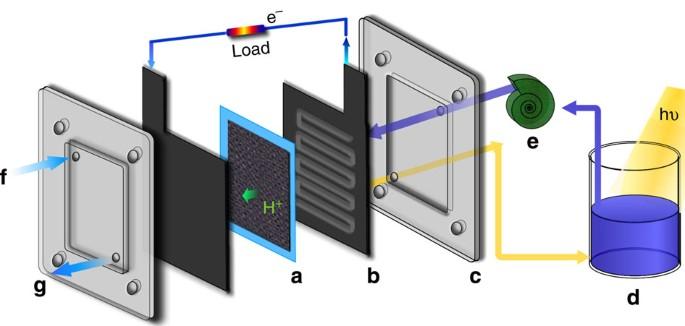Figure 1: Structure of the solar-induced hybrid fuel cell. (a) MEA (Nafion 117 polymer exchange membrane, anode made of carbon cloth and cathode loaded with Pt/C catalyst), (b) graphite bipolar plate, (c) acrylic plastic end plate, (d) transparent glass vessel with starch-H3PMo12O40(PMo12) solution, (e) pump, (f) oxygen inlet, and (g) water and oxygen outlet. Figure 1: Structure of the solar-induced hybrid fuel cell. ( a ) MEA (Nafion 117 polymer exchange membrane, anode made of carbon cloth and cathode loaded with Pt/C catalyst), ( b ) graphite bipolar plate, ( c ) acrylic plastic end plate, ( d ) transparent glass vessel with starch-H 3 PMo 12 O 40 (PMo 12 ) solution, ( e ) pump, ( f ) oxygen inlet, and ( g ) water and oxygen outlet. Full size image In this study, the photoredox process was investigated by irradiating the reaction solution under controlled temperature of 25 °C to exclude the thermal effect. It was observed that the starch–H 3 PMo 12 O 40 (PMo 12 ) aqueous solution (15 g l −1 starch and 0.3 mol l −1 PMo 12 ) gradually changes colour from the initial yellow to deep blue, which indicates the reduction of PMo 12 . 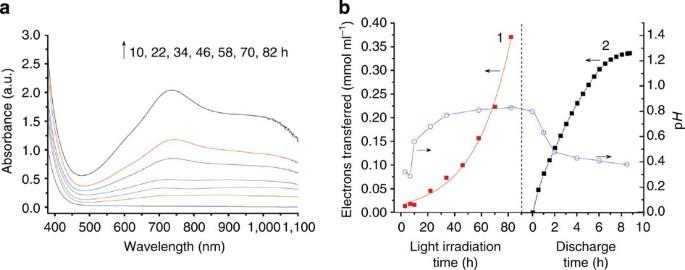Figure 2: Electron–proton transfer during photoreduction and discharge process. (a) Ultraviolet–visible spectrums of starch–H3PMo12O40(PMo12) solution under photo-irradiation (diluted to 1 mmol l−1of PMo12). (b) Number of electrons transferred and pH change plots during light irradiation and discharge period (in single cell, room temperature). Figure 2a shows the absorbance of the solution as a function of wavelength at different irradiation times. The reduced PMo 12 is known as molybdenum blue with a characteristic absorption at around 750 nm, as shown in the ultraviolet–visible spectrum. The concentration of reduced PMo 12 in the photoredox reactions was measured using spectrophotometry (calibration curve showed in Supplementary Fig. 1 ) at 750 nm and converted to the corresponding number of electrons accepted by PMo 12 . The results are plotted in Fig. 2b (curve 1). It can be seen that the electron transfer rate continuously increased during the light irradiation period. After 80 h, 0.41 mmol electrons were transferred from starch to PMo 12 per ml solution, which equals 1.23 electrons obtained per Keggin unit. Figure 2: Electron–proton transfer during photoreduction and discharge process. ( a ) Ultraviolet–visible spectrums of starch–H 3 PMo 12 O 40 (PMo 12 ) solution under photo-irradiation (diluted to 1 mmol l −1 of PMo 12 ). ( b ) Number of electrons transferred and pH change plots during light irradiation and discharge period (in single cell, room temperature). Full size image POM is not only a strong photo-oxidizing agent but also a strong Brønsted acid [17] , [18] , [19] . Under light irradiation, starch was oxidized by PMo 12 and degraded to low-molecular-weight segments, which could improve the reaction kinetics. Meanwhile, a slight increase in pH of the reaction solution during this photoredox period was observed as shown in Fig. 2b . The reason is that the addition of electrons decreases the acidity of the POM and is accompanied by protonation [17] . Therefore, POM acts as an electron and proton carrier during the photodegradation of starch. A similar behaviour has been observed and studied previously, in which the PMo 12 acted as electron-coupled-proton buffer [20] . After exposure to simulated sunlight, the starch–PMo 12 solution was cyclically pumped through the anode cell while oxygen was simultaneously fed to the cathode cell. Figure 2b (curve 2) shows the number of discharged electrons, calculated by integrating the electric current output curve. The number of electrons discharged on the electrode was 0.375 mmol electrons per ml solution, which is close to the calculated number shown in curve 1. This indicates that the electrons stored in the reduced PMo 12 were almost completely transferred to the cathode via the external circuit and captured by O 2 . After discharging, the pH was almost recovered to the original value because the oxidation of the reduced POM led to the release of protons from the POM to the solution [17] . Electron and proton transfer at elevated temperatures Molybdenum blue can strongly absorb visible-near infrared light (700–1,000 nm), which is caused by the intervalence charge transfer (CT) transitions via an oxobridge [21] . The long-wavelength light absorption leads to the conversion of light energy to thermal energy, which raises the solution temperature. As shown in Supplementary Fig. 2 , the temperature of the starch–PMo 12 reaction solution can reach up to 84 °C under actual sunlight irradiation (clear sky, 28 °C, Atlanta, GA, USA) for 90 min, which is 20.8% higher than the maximum temperature reached by deionized (DI) water exposed to the same sunlight irradiation condition. POMs can harvest electrons and protons from organics by simply heating without light irradiation as reported before [22] , [23] , [24] , [25] , [26] , [27] . Therefore, it is expected that the redox reactions between starch and PMo 12 could be further enhanced at elevated temperature. To confirm the heating effect, the starch–PMo 12 solution was heated and kept at 95 °C for 6 h without light irradiation. The transfer of electrons and change in pH of the solution during the thermal-reduction experiment are shown in Supplementary Fig. 3 , which suggest that 0.525 mmol electrons were transferred from starch to PMo 12 per ml solution by thermal degradation alone (equal to 2.13 electrons per Keggin unit). The pH value increased from 0.65 to 0.74, and then returned to 0.62 after the reduced PMo 12 solution was discharged, which is similar to the light irradiation and discharge test described previously. The results suggest that the designed biomass–POM reaction system could combine photochemical and thermal biomass degradation in a single process, which means that the sunlight utilization could be extended to the near-infrared band. Output of the starch-based cell As expected and shown in Fig. 3a , when a pure starch solution (2.5 wt%) was used alone at room temperature, the power output was very small because of the lack of catalyst on the anode to electro-oxidize the starch. When PMo 12 was added without sunlight irradiation, the power output still did not improve because the redox reaction between PMo 12 and starch could not take place at room temperature without light irradiation. PMo 12 in its original oxidation state cannot oxidize starch in the hybrid cell at room temperature without irradiation. However, after the PMo 12 was pre-reduced to molybdenum blue by the photo- or thermal-induced redox reactions with starch, power density increased to 0.28 (photo induced) and 0.44 mW cm −2 (thermal induced). The discharge process could continue for ~8 h at room temperature without light until the reduced PMo 12 in the solution was fully oxidized (evidenced by the colour change from deep blue to light yellow). 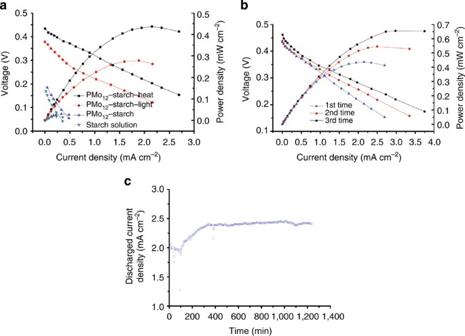Figure 3: Performances of the solar-induced hybrid fuel cell using starch as fuel. (a) Voltage–current density and power–current density plots with different reaction systems used in a single solar-induced fuel cell at room temperature; (b) plots of three repeated photo-irradiation–discharge cycles with starch–H3PMo12O40(PMo12) reaction system (discharged at room temperature); (c) current curve of continuous performance test with light irradiation at 95 °C. Figure 3: Performances of the solar-induced hybrid fuel cell using starch as fuel. ( a ) Voltage–current density and power–current density plots with different reaction systems used in a single solar-induced fuel cell at room temperature; ( b ) plots of three repeated photo-irradiation–discharge cycles with starch–H 3 PMo 12 O 40 (PMo 12 ) reaction system (discharged at room temperature); ( c ) current curve of continuous performance test with light irradiation at 95 °C. Full size image After the photo-irradiated solution was fully discharged, the solution with excess unreacted starch and its various derivatives was then exposed to simulated solar light followed by discharging again. The photo-irradiation discharge cycles were repeated three times and the power outputs were measured, as illustrated in Fig. 3b . Surprisingly, it was found that the output power density increased with the number of repeated cycles. A power density of 0.65 mW cm −2 was reached on the third cycle, even though no extra starch or PMo 12 was added. It is believed that the increase in the power density is due to the decrease in the starch molecular weight during the repeated tests. The low-molecular-weight species from oxidation and acid hydrolysis reduced the solution viscosity and increased the reaction rate with POM molecules, as compared with high-molecular-weight starch. Different from the pre-light irradiation or pre-heating tests conducted above, a continuous experiment with in-situ light irradiation and PMo 12 redox reaction simultaneous to electricity production was also conducted. The reaction solution was placed under simulated sunlight irradiation (irradiation intensity of 100 mW cm −2 ) and heated to 95 °C while being discharged simultaneously. The cell worked continuously for almost 20 h and a steady current density up to 2.5 mA cm −2 was observed, as shown in Fig. 3c . Both repeated cycle tests and in-situ continuous experiments indicate that the POM catalyst can be re-used without further treatment. Output of different biomass-based cell The solar-induced hybrid fuel cell reported in this study can be powered by various biomasses. 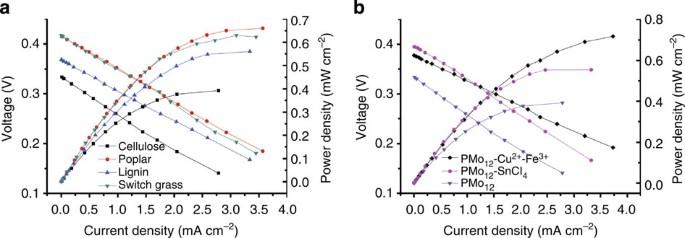Figure 4: Performances of the solar-induced hybrid fuel cell using different biomass. (a) Voltage–current density and power–current density plots of different biomasses used in the H3PMo12O40(PMo12) reaction system in photothermal experiments; (b) plots of cellulose and PMo12degradation with different metal salts as Lewis acids in photothermal experiments (discharged at room temperature). Figure 4a shows the power density that was produced by cellulose, lignin, switchgrass and poplar powder. The power density of our solar-induced hybrid fuel cell can reach 0.65 and 0.62 mW cm −2 when fueled by poplar and switchgrass powders, respectively. It should be noted that all these materials are water insoluble; hence, they were particle suspensions at the beginning, but the biomass particles were degraded and dissolved in the reaction solution as time progressed. The results illustrate that all these biomass materials can be directly used as fuel in this solar-induced hybrid fuel cell with POM as the catalyst and charge carrier. Figure 4: Performances of the solar-induced hybrid fuel cell using different biomass. ( a ) Voltage–current density and power–current density plots of different biomasses used in the H 3 PMo 12 O 40 (PMo 12 ) reaction system in photothermal experiments; ( b ) plots of cellulose and PMo 12 degradation with different metal salts as Lewis acids in photothermal experiments (discharged at room temperature). Full size image It was also noted that the power density produced by crystalline cellulose was lower than that obtained from starch solution under similar conditions, probably because of the slow hydrolysis of cellulose crystals. It was reported that some metal ions, such as Sn 4+ , Fe 3+ and Cu 2+ and so on could function as Lewis acids to help cleave glycosidic bonds in cellulose [28] , [29] . Consequently, as shown in Fig. 4b , when these promoters were used in this system, the power density obviously increased, even up to 0.72 mW cm −2 (Cu 2+ –Fe 3+ as promoters for PMo 12 ), which is almost 100 times higher than that of cellulose-based microbial fuel cells reported in literature [30] . The general principle of our solar-induced hybrid fuel cell is that PMo 12 can oxidize biomass under solar irradiation while being reduced from Mo 6+ to Mo 5+ , and then Mo 5+ can be oxidized to Mo 6+ again by oxygen through a catalytic electrochemical reaction, as illustrated in Fig. 5a . In a previous study, Yamase [31] proposed that electron transfer from organics to POM under light irradiation could result in the formation of an intermolecular charge-transfer complex. This mechanism was further investigated and accepted widely in other studies [21] , [32] , [33] . According to this mechanism, the representative reaction in our starch-PMo 12 solution is as shown in equation (1). 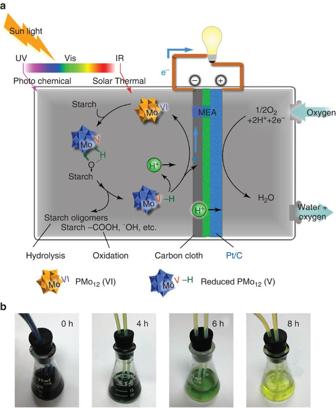Figure 5: Schematic illustration of this solar-induced fuel cell. (a) The working principle of this cell. In fact, there are 12 Mo elements in 1 POM cluster. To simplify the drawing, oxidized Mo is represented by MoVIand reduced Mo is represented by MoV, although the 12 Mo elements in the cluster may not have the same valences. (b) The colour change of starch–H3PMo12O40(PMo12) solution after electrically discharging up to 8 h. Figure 5: Schematic illustration of this solar-induced fuel cell. ( a ) The working principle of this cell. In fact, there are 12 Mo elements in 1 POM cluster. To simplify the drawing, oxidized Mo is represented by Mo VI and reduced Mo is represented by Mo V , although the 12 Mo elements in the cluster may not have the same valences. ( b ) The colour change of starch–H 3 PMo 12 O 40 (PMo 12 ) solution after electrically discharging up to 8 h. Full size image The PMo 12 has the best-known Keggin structure consisting of a central tetrahedral [PO 4 ] surrounded by 12 [MoO 6 ] octahedrons that are photosensitive [34] . Under short-wavelength light irradiation, the commonly known O→Mo ligand-to-metal CT occurs, which means the 2 p electron in the oxygen of [MoO 6 ] is excited to the empty d orbital in Mo, changing the electron configurations of Mo from d 0 to d 1 , and leaving a hole at the oxygen atom of the POM lattice [21] , [31] . This hole interacts with one electron on the oxygen atom of a hydroxyl group of starch [21] , [31] . Meanwhile, the hydrogen atom of the hydroxyl group shifts to the POM lattice to interact with the d 1 electron [21] , [31] , which is a thermally activated delocalization within the polyanion molecule [35] . Thus, the intermolecular CT complex is formed, leading to the separation of photo-excited electrons and holes, and thus stabilizing the reduced state of PMo 12 . In this study, the formed starch–PMo 12 complex was separated from the reaction solution and characterized by Fourier-transform (FT)–infrared, which provides evidence of the interaction between starch and PMo 12 (shown in Supplementary Fig. 4 and Supplementary Table 1 ). As light irradiation has a dual effect on the oxidation of biomass by POMs as verified before, both photo and heat reduction of PMo 12 can happen simultaneously in the presence of starch. As a result, POM captures an electron and proton from starch; thus, starch is oxidized and degraded to starch oligomers and glucose derivatives as shown in reaction (2). In fact, POM can accept more than one electron per Keggin unit as the reaction continued progressed, which means the increase of reduction degree of POM. It should be noted that although one Mo is reduced from VI to V valence by forming a starch–POM complex, the total charge of the polyanion (–[HPMo VI 11 Mo V O 40 ] 3− ) will not change because a proton is also transferred from starch to the POM complex at the same time. As the standard redox potential of oxygen is higher than that of the reduced POM, the Mo 5+ in the reduced PMo 12 can be oxidized at the anode by connecting to the O 2 electrode through an external circuit to produce electricity. As a result, the reduced POM (Mo 5+ ) gives one electron to the carbon anode and simultaneously releases a proton to the solution with the gradual colour change from deep blue to light yellow as shown in Fig. 5b . The electron passes through the external circuit and is captured by oxygen to form water at the cathode. At the same time, the starch molecules associated with PMo 12 are released into solution. The net effect of the above reaction is that Mo 5+ is oxidized back to Mo 6+ at the anode, and the starch is oxidized through dehydrogenation by POM catalysis. Finally, the proton diffuses to the cathode side through the proton-exchange membrane and combines with oxygen to form water. The entire discharge process is represented by reactions (3) and (4), Starch, which acts as the electron and proton donor, can be directly oxidized under light radiation or hydrolysed to small oligomers by the POM, and then continuously oxidized to a series of glucose derivatives such as aldehyde, ketones and acids, as shown in reaction (5): The direct oxidation of starch in the photochromic reaction was confirmed by FT–infrared ( Supplementary Fig. 4 ), and the degradation and further oxidation of starch glucose derivatives was verified by gel permeation chromatography ( Supplementary Fig. 5 and Supplementary Table 2 ) and 1 H, 13 C NMR analysis ( Supplementary Fig. 6 ). In addition, CO 2 is recognized as the final product in many photodegradation reactions of organic compounds by POMs [36] , [37] , [38] , and the produced CO 2 was actually detected during the operation of the solar-induced hybrid fuel cell in this study ( Supplementary Fig. 7 and Supplementary Table 3 ). As the charge carrier in this study, PMo 12 is very stable in a solution acidified by H 3 PO 4 , which was verified during our repeated cycle test using 31 P NMR analysis ( Supplementary Fig. 8 ). The performance of this solar-induced fuel cell is associated with the reduction degree and redox potential of POMs. As described before, the power density gradually increased after three repeated light irradiation–discharge cycles. Correspondingly, it was found that the reduction degree of the POM increased from 1.23 to 2.4 electrons per Keggin unit after three repeated tests. The reason for the increase in reduction degree is that low-molecular-weight oligomers and oxidized derivatives (mainly aldehydes) were formed during the photocatalytic reaction, and they have greater reduction power and higher reactivity with the POM. Therefore, with repeated light irradiation–discharge cycles, more electrons were captured by each Keggin unit, but without major changes in their chemical structures [39] , [40] . The power density of the cell is also affected by the redox potential of the POMs. As the charge carrier, POM is first reduced by oxidizing the biomass, and then the reduced POM is oxidized by oxygen. Obviously, if the standard redox potential of POM is high, it has greater tendency to oxidize the biomass but lower tendency to be oxidized by oxygen. Therefore, POMs with higher standard redox potentials are not always advantageous. In this study, three types of POMs (PMo 12 , [PW 12 O 40 ] 3− and [PV 3 Mo 9 O 40 ] 6− ) with different redox potentials [41] were used as the charge and proton carriers ( Supplementary Fig. 9 ). No simple relationship between standard redox potential of the POM and power output was observed. Faradic efficiency is considered as one important part of discharge efficiency. Faradic efficiency is defined as a ratio of the actual discharge capacity to the total electron charge transferred from the organics in the POM electrolyte solution. In this study, Faradic efficiency was as high as 91% and 94% in the discharge of the starch–PMo 12 system for photoreduction and thermal reduction, respectively ( Supplementary Fig. 10 and Supplementary Note 1 ). The solar-induced hybrid fuel cell designed in this study is a combination of solar cells, fuel cells and redox flow batteries, but has distinct differences from each. For a traditional solar cell, light energy is converted to electricity directly via the photovoltaic effect when the semiconductor or dye on the semiconductor is exposed to light. However, for our hybrid fuel cell, short-wave light excites POMs to the excited state in the presence of biomass and is stored in the form of the reduced POMs (that is, chemical energy) via the photochromic reaction. Moreover, visible and near-infrared light are absorbed by the solution and converted to heat, which can also promote the redox reaction between biomass and POM. The cell reported in this study also has a similar feature to redox flow batteries [42] in that electrolyte solutions with different valence states are used in the electrode cells. It is still different from redox flow batteries because the cathode side in our cell uses oxygen gas rather than an electrolyte solution. In addition, organic fuel is consumed in our hybrid fuel cell but no organic fuel is used in a traditional redox flow battery. The overall reaction, as discussed above, is the oxidation of organic fuel by oxygen, which is the fundamental basis of traditional fuel cells but not redox flow batteries. However, this cell is different from a traditional fuel cell [43] where catalytic reactions happen on the precious metal-loaded anode. The POM functions as a photo and thermal catalyst and charge carrier that takes electrons from biomass while reducing its own valence state to Mo 5+ under light irradiation and thermal degradation. The electrons in the POM are then transferred through the external circuit and the POM reverts to its original Mo 6+ valence state. In this study, the catalytic reactions are mediated by POM, but not on the surface of a noble metal electrode. In fact, most biomass fuels and even some artificial polymers and organic wastes can be directly degraded by the solar-induced hybrid fuel cell discussed in this study to provide electricity without using a precious metal anode. The organic impurities in crude biomass could also be oxidized as fuels, and inorganic impurities will not poison the whole process because POMs are robust and self-healing [30] . As a result, the fuels used in our solar-induced hybrid fuel cell do not have to be pure, which would significantly reduce the cost of current fuel cell technology. In essence, this solar-induced fuel cell is different from any cells or batteries reported previously, and it greatly widens the range of biomass fuels for electric power production. In summary, we demonstrated the feasibility of a new concept for fabricating a solar-induced fuel cell that directly consumes biomass fuels in the presence of a POM photocatalyst under light irradiation. Although the operation parameters have not been optimized, the power density of our solar-induced hybrid fuel can reach 0.72 mW cm −2 when cellulose was used as the fuel. Experimental details for preparation of electrolyte solution Phosphomolybdic acid (H 3 [PMo 12 O 40 ], PMo 12 ) with α-Keggin structure was purchased from TCI America. Potato starch solution (4 wt%) was obtained by cooking starch suspension for 20 min at 95 °C. Calculated amount of phosphomolybdic acid was added to the required volume of starch solution and then diluted to 20 ml total. The concentrations of PMo 12 and starch were 0.3 mol l −1 and 15 g l −1 , respectively. The starting pH of this solution was adjusted to 0.3 using concentrated phosphoric acid (85%, Alfa Aesar); thus, a clear yellow solution was obtained. Photoreducing experiment The obtained yellow solution (20 ml) was kept at a constant temperature of 25 °C using a recirculating water bath (RM6 Lauda, Brinkmann Instruments Service Inc.). Next, the reaction solution was irradiated with AM 1.5-type simulated sunlight (SoLux Solar Simulator, New York, USA; 50 W) for a certain time with a distance of 10 cm from the solution surface. The colour of the solution gradually turned from yellow to deep blue. At regular intervals, a very small amount of solution was taken out as a sample and diluted to 1 mmol l −1 PMo 12 for analysis of the concentration of reduced PMo 12 and the pH value of the solution. Thermal-reducing experiment The concentration of starch–PMo 12 solution used in this experiment was 15 g l −1 starch and 0.25 mol l −1 PMo 12 at pH 0.65. It was continuously heated under reflux at 95 °C with magnetic stirring in the dark for 6 h. The sample collection procedure was the same as that of photoreducing experiment. The prepared heteropoly blue solution was directly circulated in the designed fuel cell to generate electricity. As the phosphomolybdic blue is very stable in solution under air, this prepared solution can be stored for a long time. Analysis of electron transfer using spectrophotometry To obtain the calibration curve, pure PMo 12 solution without starch was reduced by electrochemical reduction treatment at 3 V for different times. The concentration of Mo 5+ in the PMo 12 solution (Mo 5+ and Mo 6+ mixture) was determined by titration with potassium permanganate solution (calibrated by standard sodium oxalate). Thus, the calibration curve for 1 mmol l −1 PMo 12 at different reduction degrees was obtained. The concentration of Mo 5+ in the starch–PMo 12 reaction solution was measured using the ultraviolet–visible spectrophotometer (Agilent Technologies Inc., Santa Clara, CA, USA, 8453) to calculate the amount of electrons transferred from starch to PMo 12 during light irradiation or heating. The samples taken in photoreducing or thermal-reducing experiments were diluted to a concentration of 1 mmol l −1 of total PMo 12 and then used for ultraviolet–visible measurement. Investigation of solar thermal energy transfer The experimental apparatus consisted of a polymer foam insulation system, transparent test tubes ( d =10 mm, h =175 mm) and a simulated sunlight source (SoLux Solar Simulator; 50 W) as shown in Supplementary Fig. 2b . The heteropoly blue reaction solutions were diluted to 1 and 10 mmol l −1 , and then transferred into test tubes with the same liquid levels. The simulated sunlight source was placed above the foam insulation in which the test tubes were laid side by side. The light energy density that irradiated the surface of the tubes was 100 mw cm −2 , and the temperature of the solution inside the test tubes was collected by thermocouples. In addition, the actual reaction solution (250 mmol l −1 PMo 12 ) and DI water were used in this photo-to-thermal test under actual sunlight. Assembly of solar-induced fuel cell and test methods The MEA was purchased as a commercialized product from Fuelcells Etc, TX, USA. The MEA was composed of a Nafion 117 membrane with 5 layers of carbon cloth on one side (used as the anode electrode) and 5-layer carbon cloth plus 60% Pt/C catalyst loaded at 5 mg cm −2 on the other side (used as cathode). The grain size of the active carbon used as support for the Pt/C catalyst was 74 μm and its specific surface area was 90 m 2 g −1 . The crystal size of the nano-Pt particles in the Pt/C catalyst was 4.0–5.5 nm and the specific surface area was 60 m 2 g −1 . The bipolar plates of the cell were made of high-density graphite plates with a straight flow channel 2 mm wide, 2 mm deep and 5 cm long (a total active area of 1 cm 2 ). The MEA was sandwiched between two graphite flow-field plates, which were clamped between two acrylic plastic end plates, as shown in Fig. 1 . Rubber gaskets were included on the circumference of the graphite flow-field plates to prevent any leakage. In our experiments, the prepared molybdenum blue solution was pumped through the anode reaction cell, and oxygen was flowed through the cathode cell using a compressed oxygen cylinder. The temperature of the liquid in the cell was ~25 °C (room temperature). The solution flow rate through the anode graphite plate was 12 ml min −1 and the oxygen flow rate through the cathode was 75 ml min −1 at 1 atm. A DS345 30 MHz (Stanford Research Systems) and a 4,200-SCS (Semiconductor Characterization system, Keithley Instruments Inc.) were used to examine the I – V curves using the controlled potentiostatic method. Cycling test for starch–PMo 12 system To investigate the reproducibility of this cell, three photoreduction–discharge cycles were conducted. In each cycle, the discharged fuel–PMo 12 solution was exposed to AM-1.5 simulated sunlight and kept at constant 25 °C until use. The solution was then pumped into the anode of the solar-induced fuel cell to electrically discharge for several hours over a load of 1.6 Ω resistance until the current fell below 0.1 mA. In the continuous experiments, the transparent glass vessel was placed under irradiation of AM 1.5-type simulated sunlight and heated to 95 °C during a continuous discharge experiment. The glass (sodium lime glass) was 2 mm thick, with transmission >95% for wavelengths from 320 to 1,100 nm and transmission >80% for wavelengths from 270 to 320 nm (air as blank sample, measured on Agilent Technologies 8453 ultraviolet–visible spectrophotometer). Biomasses used in the solar-induced fuel cell Crystalline cellulose was purchased from Alfa Aesar. The cellulose suspension was homogenized for 40 min to form a small particle suspension in the solution before used. Lignin was isolated from a commercial USA softwood kraft pulping liquor. Switchgrass was from Ceres, Inc. (Thousand Oaks, CA, USA) and poplar was provided by Michigan State University. These samples were washed with DI water and then dried at 45 °C over night. The dry samples were then milled in a Wiley mill through a 0.8-mm screen, yielding the biomass powder directly used in this study without any pretreatment. Different metal salts used as Lewis acids In these experiments, the reaction solutions consisted of 0.25 mol l −1 PMo 12 and 0.1 g biomass with a total solution volume of 20 ml and pH 0.5. The solution was irradiated by simulated sunlight (100 mW cm −2 ) and heated on a hotplate up to 95 °C and kept for 6 h (photothermal experiment). The discharge condition was the same as the starch–PMo 12 system. To improve the reduction degree of PMo 12 in cellulose–PMo 12 reaction system, some metal salts as Lewis acids were added. The Lewis acids used in this study include SnCl 4 (Alfa Aesar, 0.188 mol l −1 ) and Fe 3+ -Cu 2+ (Fe 2 (SO 4 ) 3 (Alfa Aesar, 0.15 mol l −1 ); CuSO 4 (Alfa Aesar, 0.15 mol l −1 ). Different POMs used in this hybrid fuel cell Three different POMs with various electrode potentials were used in this study: PMo 12 , phosphotungstic acid and vanadium substituted phosphomolybdic acid. Phosphotungstic acid (H 3 [PW 12 O 40 ]) was purchased from Sigma-Aldrich, and vanadium-substituted phosphomolybdic acid (H 6 [PMo 9 V 3 O 40 ]) was synthesized by the method in reported literature [41] . In comparison experiments, the reaction solutions consisted of 0.25 mol l −1 POMs, 0.3 g starch and a total solution volume of 20 ml at pH 0.5. The solution was irradiated by simulated sunlight and heated at 95 °C for 6 h (that is, photothermal experiment). For comparison, phosphotungstic acid was fully reduced by ascorbic acid (1:1 molar ratio) in solution under light irradiation and heating at 95 °C. The discharge conditions were the same as described above. Product analysis of starch degradation The starch–PMo 12 complex was separated through precipitation from the photoredox reaction system by salting out (excess Na 2 SO 4 ). The sample was then filtered and dried in a vacuum drying chamber at 30 °C overnight. The changes in the starch that was associated with PMo 12 were characterized by FT–infrared. FT–infrared spectra were obtained by averaging 64 scans from 4,000 to 650 cm −1 with 4 cm −1 resolution. Gel permeation chromatography was used to determine the changes in molecular weight of starch. Samples were taken from the reaction solution at different times and the proper amount of NaOH solution was added. The PMo 12 degraded to MoO 4 2− in alkaline solution and the final concentration of organic substance was around 1 mg ml −1 with pH 10. The analysis was performed on an Agilent 1,200 HPLC System (Agilent Technologies Inc.) equipped with ultrahydrogel columns (Waters Corporation, Milford, MA, USA) and an Agilent RI detector using DI water as the mobile phase (0.5 ml min −1 ) with injection volumes of 25 μl. 1 H NMR and 13 C NMR were used to analyse the final products of starch in the solution. To increase the signal intensity, light irradiation and discharge cycles were repeated four times. The starch–POM solution after repeated irradiation and discharge was dried at 80 °C in vacuum, then resolved in D 2 O for the NMR. 1 H and 13 C NMR spectral data reported in this study were recorded with a Bruker Avance/DMX 400 MHz NMR spectrometer. Quantitative 13 C NMR employed an inverse gated decoupling pulse sequence, 90° pulse angle, a pulse delay of 5 s and 6,000 scans. Quantitative 1 H NMR was acquired with 16 scans and 1 s pulse delay. To collect and analyse the emission gas in the hybrid fuel cell, an airtight glass vessel was connected with an emission gas outlet and a valve (shown in Supplementary Fig. 7 ). The starch–PMo 12 solution (15 g l −1 starch and 0.3 mol l −1 PMo 12 ) was stored in the airtight glass vessel and exposed to simulated sunlight (100 mW cm −2 ) and kept at 95 °C. Meanwhile, the starch–PMo 12 solution was pumped to the anode chamber of the fuel cell and discharged for 3 days. A gas collection bag was connected to the gas outlet through a rubber tube. The composition of gas was analysed on Varian 490 micro-GC equipped with a Pora Plot U (10 m) column. 31 P NMR was used to analyse the stability of POM. After several repeated irradiation and discharge cycles, the reaction solution was dried at 95 °C then resolved in D 2 O for 31 P NMR. The spectral data were collected on a Bruker Avance/DMX 400 MHz NMR spectrometer with 8 s pulse delay. How to cite this article: Liu, W. et al . Solar-induced direct biomass-to-electricity hybrid fuel cell using polyoxometalates as photo-catalyst and charge carrier. Nat. Commun. 5:3208 doi: 10.1038/ncomms4208 (2014).